Novel polymer-free iridescent lamellar hydrogel for two-dimensional confined growth of ultrathin gold membranes Hydrogels are generally thought to be formed by nano- to micrometre-scale fibres or polymer chains, either physically branched or entangled with each other to trap water. Although there are also anisotropic hydrogels with apparently ordered structures, they are essentially polymer fibre/discrete polymer chains-based network without exception. Here we present a type of polymer-free anisotropic lamellar hydrogels composed of 100-nm-thick water layers sandwiched by two bilayer membranes of a self-assembled nonionic surfactant, hexadecylglyceryl maleate. The hydrogels appear iridescent as a result of Bragg’s reflection of visible light from the periodic lamellar plane. The particular lamellar hydrogel with extremely wide water spacing was used as a soft two-dimensional template to synthesize single-crystalline nanosheets in the confined two-dimensional space. As a consequence, flexible, ultrathin and large area single-crystalline gold membranes with atomically flat surface were produced in the hydrogel. The optical and electrical properties were detected on a single gold membrane. Recently, the research on hydrogels has been paid great attention as their flexible and tunable properties [1] (for example, response to the external stimuli) and wider applications (for example, gel electrophoresis, chemical sensing, drug delivery, as a biointerface, and as actuators) [2] , [3] , [4] , [5] , [6] . Hydrogels, consisting of polymers or small organic molecules, are generally thought to be formed by three-dimensional, elastic networks whose interstitial spaces are filled with water [7] . Basically, most of the gelation phenomenon arises from the formation of nano- to micrometer- scale fibres or polymer chains either physically branched (in the form of interconnected network) or entangled with each other to trap water via surface tension [8] . Unlike polymer gels where fibres/discrete polymer chains are formed by strong chemical bonds, the strands of small molecule hydrogels are assembled by noncovalent weak interactions that enable small molecule hydrogels thermally reversible [9] . In contrast to the conventional isotropic hydrogels with fibre/polymer chains-based network, a few of anisotropic hydrogels with one-dimensional periodic lamellar structure have been discovered and received particular attentions, which expand our understanding and knowledge about hydrogels [10] , [11] , [12] . A lamellar biological hydrogel comprised of fluid membranes of lipids and surfactants with small amounts of poly(ethylene glycol)-derived polymer lipids was firstl reported by C. R. Safinya et al. [10] The lamellar hydrogel with the maximum water spacing of ~40 nm between adjacent layers exhibits birefringent liquid crystalline behaviour. As for the origin of the anisotropic hydrogels, the introduction of poly(ethylene glycol)-derived polymer lipids has been considered to be essential. It is because that PEG-lipid segregation, formed at the high curvature regions of lipid membranes, prevents the water flowing and finally forms the gel phase. Such kind of lamellar structures was then extended to the fabrication of photonic hydrogels by introducing a soft polymer hydrogel into the interlamellar spacing [11] . Recently, an interesting lamellar hydrogel made of a polyelectrolyte-containing block polymer was reported to be a broad-wavelength-range responsive photonic crystal with tunable layer thickness [12] . The gelation of this hydrogel is essentially driven by the nature of swellable polymer network of polyelectrolyte block. Strictly speaking, these anisotropic hydrogels with lamellar structures require the assistance of various polymers at all events. Here we report a polymer-free lamellar hydrogel composed of 100-nm-thick water layers sandwiched by two bilayer membranes that consist of a self-assembled nonionic surfactant hexadecylglyceryl maleate (HGM) and a tiny amount of co-surfactant sodium dodecyl sulphonate (SDS). The synthesized hydrogel appears of blue–violet colour as a result of Bragg’s reflection of visible light from the periodic lamellar plane. This particular lamellar hydrogel with an extremely wide water spacing is used as a soft two-dimensional (2D) template to direct the growth of 2D single-crystalline membranes. As the diffusion of reactive precursor ions is slowed down to a certain extent and the reaction is effectively constrained in the confined 2D space, flexible, ultrathin (3.6 nm in thickness) and large area (>100 μm 2 ) single-crystalline Au membranes with atomically flat surface can be produced in the hydrogel. The optical and electrical properties of a single Au membrane are detected, which exhibit the characteristic of 2D nanomaterials. Characterization of HGM hydrogel Iridescent solution formed from dilute aqueous solutions of some kind of surfactants where lamellar bilayer membranes are separated uniformly by water with equal distances on the order of the light wavelength has been investigated as early as 1,938 (ref. 13 ). As a typical example, iridescent dodecylglyceryl itaconate (DGI) solution made of a nonionic surfactant, DGI was firstly developed by Satoh and Tsujii [14] . HGM, as a derivative of DGI, could form lamellar bilayer membranes and also generate iridescent solution at the temperature above its Krafft point (37 °C) ( Supplementary Fig. 1 ). The single and uniform colour throughout the system indicates the formation of an ordered structure consisting alternate HGM bilayers and water layers with a periodic distance on the order of submicrometers throughout the whole system following the Bragg’s equation (2 nd sin θ = λ , where n , d , θ and λ are the refractive index of water, the periodic spacing, the angle of incidence and the wavelength of the reflected light, respectively) ( Fig. 1 ). It is worthy to note that the colour of HGM solution is angle-dependent structure colour ( Supplementary Fig. 2 ). Although HGM system is composed of polydomains of lamellar structure, these polydomains are prone to be uniaxially oriented owing to shear force between the wall of container and solution ( Supplementary Fig. 2a ) under our special treatment on the system. This uniaxial orientation can be also observed in the scanning electron microscopy image of HGM hydrogels after freeze-drying treatment ( Supplementary Fig. 3 ). Such a treatment was often used by other researchers to unidirectionally align lamellar structure [11] . Different from DGI, the HGM system has the unique thermal responsibility. 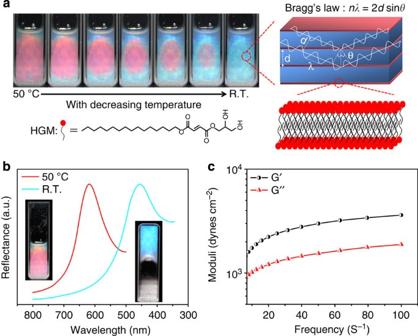Figure 1: Colour and structure characterization of HGM hydrogel. (a) Colour change of HGM solution with decreasing temperature and corresponding schematic of HGM hydrogel with alternative structure of HGM lamellar bilayer and water layer. (b) Reflection spectra of HGM solution at 50 °C and room temperature and their photographs correspondingly. (c) Dynamic elastic moduli of HGM hydrogel as a function of frequency. The larger elastic storage modulus G′ than viscous loss modulus G′′ in a wide range of frequency indicates a typical characteristic of gel. Figure 1a shows the photographs of iridescent HGM solution with HGM concentration of 1.6 wt% with the decreasing of temperature from 50 °C to room temperature. It clearly shows that the colour of the solution shifts from red to shinning blue, gradually. With the colour change, the state of HGM system changes from liquid to gel (inset in Fig. 1b ). The reflection spectrum was used to characterize the ordered structure with periodical distance of the order of sub-micrometre and analysis interlayer spacing. As shown in Fig. 1b , the HGM solution shows a peak at 618 nm when the temperature is 50 °C, which corresponds to the periodic spacing between adjacent HGM bilayer of 235 nm calculated by the Bragg’s equation. For HGM hydrogel at room temperature, the peak shifts to 455 nm, corresponding to the periodic spacing of 173 nm. The 163-nm blue shift indicates that small amount of water is squeezed out from the interlayer of HGM bilayer during the transition of HGM solution from liquid to gel phase. The dynamic rheology test on the gel sample was done by measuring the real (storage elasticity modulus, G ′) and imaginary (viscous loss modulus, G ′′) parts of the dynamic moduli as a function of frequency. Over the frequency range, G ′ is substantially greater than G ′′ ( Fig. 1c ), representing a typical characteristic of gel. Figure 1: Colour and structure characterization of HGM hydrogel. ( a ) Colour change of HGM solution with decreasing temperature and corresponding schematic of HGM hydrogel with alternative structure of HGM lamellar bilayer and water layer. ( b ) Reflection spectra of HGM solution at 50 °C and room temperature and their photographs correspondingly. ( c ) Dynamic elastic moduli of HGM hydrogel as a function of frequency. The larger elastic storage modulus G′ than viscous loss modulus G′′ in a wide range of frequency indicates a typical characteristic of gel. Full size image Reflection spectra with different HGM concentrations As for a uniform iridescent solution in a low-surfactant concentration around 1–2 wt%, the thickness of water layer d , is directly relevant to the surfactant weight percentage c , following the relationship as below: where ρ 1 and ρ 2 are the densities of surfactant and water layer, respectively, and d 1 is the thickness of surfactant layer [15] . It shows that d is in proportion to (1− c )/ c . The same correlation is also observed in HGM solution. 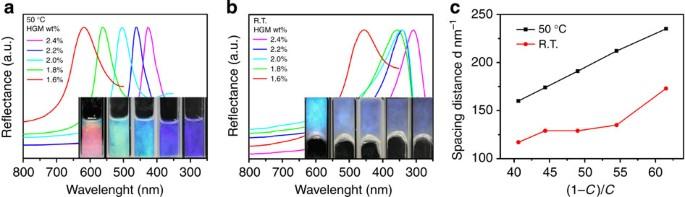Figure 2: Reflection spectra with different HGM concentrations. (a) Reflection spectra of HGM solutions at 50 °C. (b) Reflection spectra of HGM hydrogels at room temperature. (c) Plot of water layer thickness (dspacing) versus (1−c)/c(cis HGM weight fraction). Figure 2a shows the reflection spectra of iridescent HGM solutions with different HGM concentration. With increasing concentration of the surfactant from 1.6 to 2.4 wt%, the wavelength of the maximum reflection changes from 618 nm in case of 1.6 wt% to 426 nm in case of 2.4 wt%. Correspondingly, the colour of the solutions changes from red to blue (inset in Fig. 2a ). Cooling these HGM solutions to room temperature, all the solutions become iridescent hydrogels and the colour of the hydrogels appears from dim blue to light blue with the increase of HGM concentration correspondingly (inset in Fig. 2b ). The reflection spectra of the hydrogels still exhibit strong and sharp peaks, although obvious blue shifts of their reflection peaks are observed as compared to HGM solutions ( Fig. 2b ). It indicates that the uniform lamellar structures are well maintained in the hydrogel system. The spacing d , for every sample, could be calculated from the Bragg’s equation based on its maximum reflection wavelength. For both HGM solutions and hydrogels, the obtained d spacings against (1− c )/ c are plotted, respectively, as shown in Fig. 2c . It can be seen that the plot for HGM solutions is a straight line, which fits well to the above equation. It indicates that the highly homogeneous lamellar structure exists in every HGM solution, and almost no free water and excessive HGM molecules exist out of the lamellar structures. However, the plot for HGM hydrogels shows a little deviation from the above equation. This result suggests that defects more or less are formed in HGM hydrogel, although the whole-hydrogel system maintains periodically ordered structure from the overall point of view. Figure 2: Reflection spectra with different HGM concentrations. ( a ) Reflection spectra of HGM solutions at 50 °C. ( b ) Reflection spectra of HGM hydrogels at room temperature. ( c ) Plot of water layer thickness ( d spacing) versus (1− c )/ c ( c is HGM weight fraction). Full size image The freeze-fracture electron microscopy was employed further to examine the microstructures of HGM solution ( Fig. 3a ) and HGM hydrogel ( Fig. 3b ). The image of HGM solution is filled with well ordered, parallel and gently waving lamellae, spanning microns. Almost no defects are observed in the entire view. This image is consistent with the periodically ordered lamellar structure as we expected for iridescent solution system. As for HGM hydrogel, the lamellae become more curved and the defects in terms of two opposite-edge dislocations occasionally appear. Two structure models are drawn to illustrate the difference between the two phases on the level of molecular arrangement. In HGM solution, co-surfactant SDS embeds in the planar HGM bilayer membrane evenly to provide repulsive interaction between two lamellae against the thermal undulation. As temperature decreases, the planar lamellae are prone to curl to be more thermodynamically stable. The edge-dislocation defects are thus generated in HGM hydrogel. The defect regions are stabilized by the segregation of SDS molecules to compensate the high-membrane curvature. As for a surfactant, its preferred packing structure in solution is determined by the critical packing parameter (CPP), which is the ratio of effective volume v , head group area a 0 and chain length l c (CPP= v/a 0 l c ) [16] , [17] , [18] , [19] , [20] . The HGM molecule has similar area of head group and tail with CPP ~1. It is favourable to form planar bilayer structure. The SDS molecule has an obviously larger head group area than tail area with CPP ~0.33. Its preferred phase in water is vesicle. From this point of view, it is reasonable to propose that with the occurrence of curvature-induced in-plane phase separation with temperature decreasing, SDS molecules with natural radius concentrate in the regions of high-membrane curvature to stabilize the edge-dislocation defects. The formation of the edge-dislocation defects thus increases the viscoelasticity of the HGM system because the defects could resist the water flow along the direction normal to the membranes layers. Although only a small amount of edge-dislocation defects are generated and verified by freeze-fracture electron microscopy observation, it is believed to be the origin of hydrogel. 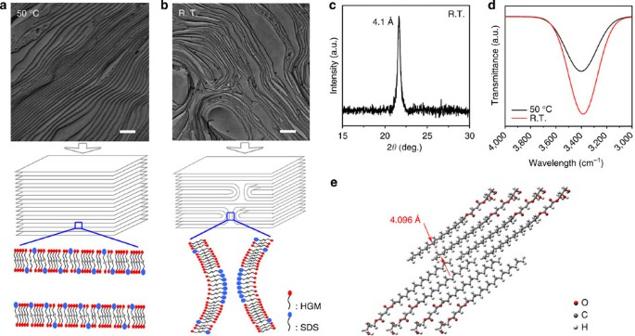Figure 3: Microstructure analysis of HGM hydrogel. Freeze-fracture electron microscopy images of HGM solution (1.6 wt%) at 50 °C (scale bar, 1 μm) (a) and at room temperature (scale bar,1 μm) (b), and their corresponding schematic showing the arrangement of HGM and SDS molecules. (c) X-ray diffraction pattern of HGM hydrogel (1.6 wt%) at room temperature. (d) Fourier transform infrared spectra of HGM solutions (1.6 wt%) at 50 °C and at room temperature. (e) The optimal packing structure of HGM lamellar bilayer membrane obtained by modelling with Forcite module. Figure 3: Microstructure analysis of HGM hydrogel. Freeze-fracture electron microscopy images of HGM solution (1.6 wt%) at 50 °C (scale bar, 1 μm) ( a ) and at room temperature (scale bar,1 μm) ( b ), and their corresponding schematic showing the arrangement of HGM and SDS molecules. ( c ) X-ray diffraction pattern of HGM hydrogel (1.6 wt%) at room temperature. ( d ) Fourier transform infrared spectra of HGM solutions (1.6 wt%) at 50 °C and at room temperature. ( e ) The optimal packing structure of HGM lamellar bilayer membrane obtained by modelling with Forcite module. Full size image Our polymer-free lamellar hydrogel composed of wide and periodic water spacing up to 173 nm (which corresponds to water content of 98.4 wt%) is different from the previous work [10] . The special structure of HGM hydrogel is beyond the common sense of lamellar-based hydrogel, which allows us to explore the key factors to sustain such structure from the viewpoint of molecular arrangement and intermolecular force. It is generally accepted that the lamellar bilayer membrane system usually experiences two stable phases around Krafft point [21] , [22] . Above Krafft point, it presents in the form of lamellar liquid crystalline phase showing iridescent colour. When the temperature is below Krafft point, the system transforms to be an anhydrous crystal, identified as β-crystalline state ( L β , often called the ‘coagel’). The coagel state does not remain the characteristic of iridescent solution but becomes an isotropic system. The driving force for the transformation from lamellar liquid crystalline phase to L β phase is believed to be the strong intermolecular hydrogen bonds established between the head groups of in-plane molecules at L β phase state. It usually gives rise to a spacing of adjacent molecules around 4.5–4.6 Å according to previous reports [21] , [22] . Besides the two phases, there is an intermediate phase called α-crystalline phase ( L α ), which is metastable and readily transforms to L β phase. The main characteristic of L α phase is thought to be a hexagonal molecule packing in one layer with a spacing of adjacent molecules around 4.1–4.2 Å. Different from the commonly reported lamellar bilayer membranes, in our HGM system, L α phase is a very stable state and it could be maintained below Krafft point even when the temperature approaches 0 °C, which can be directly verified by its stable iridescent colour with the temperature decreasing. The X-ray Diffraction of HGM hydrogel exhibits a sharp and strong diffraction peak ( Fig. 3c ) that corresponds to a 4.1-Å spacing of adjacent HGM molecules. This value is consistent with the characteristic spacing of L α phase. To further confirm the rationality of such packing, Forcite with the Dreiding force field and Gasteiger charges are used to optimize the packing of HGM molecules. As shown in Fig. 3e , the result of theoretical calculation also indicates the optimized spacing of HGM molecules at 4.096 Å. From the above discussions, we know that the transformation from lamellar liquid crystalline phase to L β phase is accompanied by the formation of intermolecular hydrogen bonds. To characterize the intermolecular interaction, Fourier transform infrared spectra of HGM solution and HGM hydrogel were recorded as shown in Fig. 3d . There is only one peak at 3,404 cm −1 in both of the two spectra. This peak corresponds to the hydrogen bonding between HGM and water, and no peaks corresponding to the hydrogen bonding formed by intermolecular HGM are observed [23] . It reveals that HGM prefers to form hydrogen bond with water rather than with HGM molecules. Therefore, it is speculated that owing to weak hydrogen bonding among HGM molecules, the transformation from lamellar liquid crystalline phase to L α phase occurs but further crystallization from L α to L β gel does not. These results provide solid evidence for our description and understanding of HGM hydrogel. HGM hydrogel composed of periodically ordered sandwich structure of 100-nm-thick water layers and lamellar bilayer membranes could serve as ‘soft templates’ to direct the growth of ultrathin single-crystalline Au nanosheets. The synthesis of Au nanosheets was carried out by directly introducing a certain amount of chloroauric acid (HAuCl 4 ) as precursor into HGM hydrogel with the concentration of 1.6 wt%. The two hydroxyl groups at the hydrophilic end of each HGM molecule can function as weak reductants to reduce HAuCl 4 dispersed in the water layer to Au. Ultrathin Au nanosheets with ultralarge area (>100 μm 2 ) are prepared in the hydrogel system ( Fig. 4a,b ). Interestingly, owing to their extremely small thickness, the nanosheets are flexible and form into a curled shape like a thin polymer membrane or graphene. We, therefore, call the Au nanosheets membranes. A high-resolution transmission electron microscopy image taken from a typical Au membrane reveals that it is a single crystalline with a fringe spacing of 0.24 nm ( Fig. 4c ). The presence of the forbidden 1/3(422) reflection indicates that the surface of the Au sheet is atomically flat [24] . The corresponding selected-area electron diffraction pattern ( Fig. 4c inset) clearly shows the single-crystalline characteristic of Au, and the hexagonal diffraction spots indicate it to be highly (111)-oriented. The thickness distribution of Au membranes statistically analysed by atomic force microscopy measurement gives a narrow thickness distribution around 5–6 nm ( Supplementary Fig. 4 ). 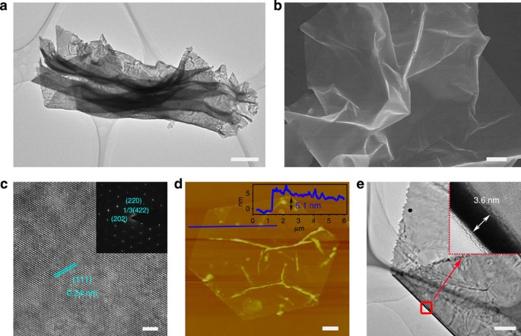Figure 4: Morphology and structure of and ultrathin Au membrane. (a) Transmission electron microscopy (scale bar, 1 μm), (b) Scanning electron microscopy (scale bar, 1 μm), and (c) High-resolution transmission electron microscopy images (scale bar, 2 nm) and (inset) selected-area electron diffraction pattern of a typical Au membrane. (d) Topological atomic force microscopy image (scale bar, 1 μm) and (inset) height profile of a typical Au membrane showing the thickness of 5.1 nm. (e) Transmission electron microscopy image (scale bar, 200 nm) and (inset) enlarged image taken at the folded edge of a typical Au membrane where the naked thickness of the Au membrane is obtained by measuring the width of the folded edge to be 3.6 nm. Figure 4d is the atomic force microscopy image of a typical Au membrane with a thickness of 5.1 nm as shown in the corresponding height profile curve. In fact, owing to the adsorption of HGM molecules on Au membrane surface, this value should not be the thickness of naked Au membrane. The real thickness of Au membrane is obtained to be 3.6±0.5 nm by measuring the width of folded edges of an Au membrane ( Fig. 4e ). This method has been well used to effectively distinguish monolayer from bilayer sheets of graphene [25] and characterize the thickness of gold sheets [26] . The extra ~1.5 nm is ascribed to the layer of HGM adsorbed on Au surface. The synthesis of ultrathin nanocrystals of nonlayered materials is of scientific significance yet very hard via a wet chemical route because of the lack of methods of inducing anisotropic growth in 2D structure. The unique HGM lamellar hydrogel with 100-nm-thick water layers has demonstrated its effectiveness and provides a powerful soft 2D template for producing 2D nanomaterials of nonlayered structure. Both theoretical and experimental results have demonstrated that the viscosity of water increases in the confined 2D space in extended nanoscale [27] , [28] , [29] . In HGM hydrogel, the diffusion of reactive ions is slowed down greatly and constrained in the confined 2D space, which effectively decreases the growth rate of Au, especially in the direction vertical to the HGM bilayer membrane. It is thus benefit for controlling the thickness and growth orientation ( Supplementary Fig. 5 ). Figure 4: Morphology and structure of and ultrathin Au membrane. ( a ) Transmission electron microscopy (scale bar, 1 μm), ( b ) Scanning electron microscopy (scale bar, 1 μm), and ( c ) High-resolution transmission electron microscopy images (scale bar, 2 nm) and (inset) selected-area electron diffraction pattern of a typical Au membrane. ( d ) Topological atomic force microscopy image (scale bar, 1 μm) and (inset) height profile of a typical Au membrane showing the thickness of 5.1 nm. ( e ) Transmission electron microscopy image (scale bar, 200 nm) and (inset) enlarged image taken at the folded edge of a typical Au membrane where the naked thickness of the Au membrane is obtained by measuring the width of the folded edge to be 3.6 nm. Full size image To our knowledge, the Au membranes fabricated by us are the thinnest single-crystalline Au sheets in micrometre scale reported so far. To demonstrate their 2D characteristic, transparency ( Supplementary Fig. 6 ) and electrical conductivity properties of a single Au membrane are examined as shown in Fig. 5 . The transmittance spectrum recorded on an ~5-nm -thick Au membrane shows that its transparency is as high as 83% at 550 nm ( Fig. 5a ), which is consistent with theoretical simulation of the transmittance of a single-crystalline Au film with similar thickness based on the dielectric constant of bulk Au [30] . Electrical conductivity was measured by drop-casting Au membrane onto the gold electrodes with a 10-μm gap (inset in Fig. 5b ). After annealing the Au membrane-bridged electrode at 400 °C for 4 h to eliminate the contact resistance as much as possible ( Supplementary Fig. 7 ), I–V curve was monitored with a Keithley 2602 Source Metre at ambient condition as shown in Fig. 5b . The straight line corresponds to the resistance of 16 Ω for such a thin Au membrane. The resistivity of the Au membrane has been calculated to be 4.0 × 10 −8 Ωm. This value is comparable to the corresponding Au value (ρ bulk =2.2 × 10 −8 Ωm) and epitaxial Au films [31] and is 1–2 orders of magnitude lower than the thermally evaporated Au film [32] . It indicates that our ultrathin Au membrane possess good conductivity. These results suggest that the ultrathin and large-size Au membranes have potential applications for next-generation transparent and conducting electronic devices. 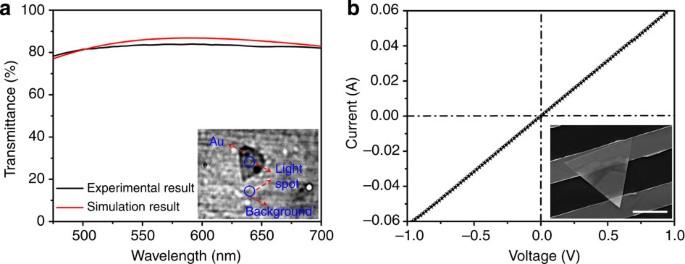Figure 5: Transmittance and electrical conductivity of an ultrathin Au membrane. (a) Transmittance spectra of an ~5-nm -thick Au membrane: experimental result (black line) and theoretical simulation result (red line). The inset is an optical image of Au membrane on glass substrate. The two circles are marked to indicate the position of light spot on Au membrane and on glass substrate as background, respectively. (b) I–V curve of an ~5-nm-thick Au membrane spanning two gold electrodes with a distance of 10 μm. The inset is the optical image of the device (scale bar, 10 μm). The thickness of the Au membranes was confirmed by AFM measurement. Figure 5: Transmittance and electrical conductivity of an ultrathin Au membrane. ( a ) Transmittance spectra of an ~5-nm -thick Au membrane: experimental result (black line) and theoretical simulation result (red line). The inset is an optical image of Au membrane on glass substrate. The two circles are marked to indicate the position of light spot on Au membrane and on glass substrate as background, respectively. ( b ) I–V curve of an ~5-nm-thick Au membrane spanning two gold electrodes with a distance of 10 μm. The inset is the optical image of the device (scale bar, 10 μm). The thickness of the Au membranes was confirmed by AFM measurement. Full size image In conclusion, we discovered special polymer-free iridescent lamellar hydrogels formed from surfactants solely. Unlike common hydrogels that consist of fibres/discrete polymer chains-based network, the anisotropic hydrogel with one-dimensional periodic lamellar structure has extremely thick water layer up to sub-micrometre scale sandwiched by lamellar bilayer membranes of a self-assembled HGM molecule. The origin of hydrogel is ascribed to the formation of certain amount of edge-dislocation defects derived from curved bilayer membranes, which effectively restrain the flow of water. The particular lamellar hydrogel was used as a soft 2D template to guide the growth of 2D single-crystalline Au sheets. Free-standing, ultrathin and ultralarge single-crystalline Au membranes with atomically smooth surface were successfully synthesized, and exhibited interesting optical and electrical properties. The unique hydrogel system with highly ordered water layers opens a new way for producing various 2D nanomaterials and its abundant water/biomembrane interfaces are very promising to be used in bio-related field. Chemicals 1-Hexadecanol (CH 3 (CH 2 ) 14 CH 2 OH, 98%; Alfa), Maleic anhydride (95%, Sigma-Aldrich), Glycidol (96%, Sigma-Aldrich), Hydrogen tetrachloroaurate(III) hydrate (HAuCl 4 , 99.9% (metals basis), Au 49% min; Alfa), Sodium dodecyl sulphate (CH 3 (CH 2 ) 10 CH 2 OSO 3 Na, ACS reagent, ≥99.0%; Sigma-Aldrich), Ethyl alcohol absolute (CH 3 CH 2 OH, ≥99.7%; Sinopharm Chemical Reagent), n-hexane (CH 3 (CH 2 ) 4 CH 2 OH, AR, Sinopharm Chemical Reagent), Acetic ether (CH 3 COOCH 2 CH 3 , AR, Sinopharm Chemical Reagent), Acetone (CH 3 COCH 3 , AR, Sinopharm Chemical Reagent) Deuterochloroform (CDCl 3 , Sinopharm Chemical Reagent) were used without further purification. Millipore deionized water was used in this work. Synthesis of HGM HGM was synthesized according to previous report [33] . In detail, Maleic anhydride (21.56 g, 0.22 mol) was mixed and reacted with hexadecanol (52.12 g, 0.215 mol) at 116 °C for 1 h to obtain hexadecyl maleate. After the reaction was completed, 50 ml of hexane was added to the above mixture at 80 °C under a vigorous mechanical stirring and the crude product of white crystal was precipitated. The crude sample of hexadecyl maleate was recrystallized from ethanol. The melting point of the purified sample was 69–71 °C. The obtained hexadecyl maleate (11.56 g, 0.034 mol) was dissolved in toluene (10 ml) and reacted with glycidol (7.5 g, 0.102 mol) at 108 °C in the presence of 20 mg (39.7 μmol) pyridinium p-toluenesulphonate as a catalyst. The mixture was refluxed with stirring for 5 h at 108 °C. The toluene was evaporated under reduced pressure. The crude product was applied to a silica-gel column and eluted with a hexane/ethyl acetate mixture (3/2 by volume). The collected HGM fraction was purified twice by recrystallization from an acetone/hexane mixture (1/1 by volume). Nuclear magnetic resonance analysis ( Supplementary Fig. 8 ) shows that the purity of the final product (mp. 50–52 °C) is more than 99%. Synthesis of ultrathin Au membrane In the typical preparation of ultrathin gold membrane, the iridescent solution of HGM with concentration of 1.6 wt% was prepared at 55 °C for 1 day to get a stable and uniform phase of lamellar structure. To obtain the large, ultrathin and single-crystal gold membrane, we mix the HGM solution (2 ml) with 3.2 μmol aqueous chloroauric acid, followed by blending the mixture solution mildly to a homogeneous solution. The ordered structure of original HGM solution is well maintained under this condition, which has been confirmed by reflection spectrum. Then we put the reaction bottle in an ambient environment at room temperature for 1 day. After that, a mass of large Au membranes was obtained. The Au membranes were then washed at least three times with ethanol and chloroform, respectively, before further characterization. Freeze-fracture transmission electron microscopy experiment The typical processes were as follows: HGM solutions were kept in a water bath for 1 day to obtain the equilibrium state. A certain amount of a sample was dropped in the specimen carrier and frozen by liquid nitrogen. The frozen samples were then fractured at −120 °C in a JFD-9010 vacuum chamber. After treating by etching at −90 °C, the samples were tilted and coated by platinum and carbon, subsequently. The replicas were peeled off after melting the samples in ambient conditions. Transmission electron microscopic observation was made on a Tecnai G2 F20 S-Twin field-emission transmission electron microscope. Theoretical simulation of the transmittance of Au membrane Here we consider a homogenous Au membrane with thickness of h , illuminated by normally incident light with the wavelength λ . By applying the boundary conditions at each boundary of the membrane, the reflection and transmission coefficients r and t , respectively, can be expressed as and with β =2π n 2 h / λ , and the Fresnel coefficients r ij , t ij given by and the reflectivity and transmissivity are given by and (ref. 34 ). Here the subscripts i,j =1, 2, 3 refer to the three media: air, Au and air ,respectively, and their refractive indices are set as n 1 = n 3 =1.0, , respectively. The frequency-dependent Au dielectric constant ε Au was obtained by using the Drude-Lorents model as reported in previous work [35] . Characterization Scanning electron microscopy images were obtained on a field-emission scanning electron microscope (Hitachi S4800, Japan). Transmission electron microscopy was measured on a Tecnai G2 F20 S-Twin field-emission transmission electron microscope. X-ray Diffraction was collected on a Bruke D8. Atomic Force Microscopy was obtained on a Dimension 3100, Veeco. Transmittance of single Au nanomembrane was measured on Laica DMI3000 M. Reflection spectra were measured by a UV/Vis spectrometer (PerkinElmer, Lambda 750) with the fixed incident angle of 83°. How to cite this article: Niu, J. et al. Novel polymer-free iridescent lamellar hydrogel for two-dimensional confined growth of ultrathin gold membranes. Nat. Commun. 5:3313 doi: 10.1038/ncomms4313 (2014).